Spatial mapping of multimode Brownian motions in high-frequency silicon carbide microdisk resonators High-order and multiple modes in high-frequency micro/nanomechanical resonators are attractive for empowering signal processing and sensing with multi-modalities, yet many challenges remain in identifying and manipulating these modes, and in developing constitutive materials and structures that efficiently support high-order modes. Here we demonstrate high-frequency multimode silicon carbide microdisk resonators and spatial mapping of the intrinsic Brownian thermomechanical vibrations, up to the ninth flexural mode, with displacement sensitivities of ~7−14 fm Hz −1/2 . The microdisks are made in a 500-nm-carbide on 500-nm-oxide thin-film technology that facilitates ultrasensitive motion detection via scanning laser interferometry with high spectral and spatial resolutions. Mapping of these thermomechanical vibrations vividly visualizes the shapes and textures of high-order Brownian motions in the microdisks. Measurements on devices with varying dimensions provide deterministic information for precisely identifying the mode sequence and characteristics, and for examining mode degeneracy, spatial asymmetry and other effects, which can be exploited for encoding information with increasing complexity. The concept of exploiting resonance modes in mechanical systems for generating and processing high–frequency (HF) signals has profoundly facilitated scientific studies [1] , [2] , [3] , [4] and accrued successful enterprises in radio engineering, communication and sensing technologies [3] , [5] , [6] , [7] . At device level, fundamental approaches involve manipulating flexural vibrations of mechanical structures (for example, tuning forks) and acoustic waves in crystals (for example, quartz), harnessing the sharply frequency-selecting functions offered by the high-quality ( Q ) resonances in these vibrations and waves [1] , [2] , [3] , [4] , [5] , [6] , [7] . Advances in surface micro/nanomachining technologies [8] , [9] have spurred unceasing miniaturization of vibrating mechanical devices, with rapid developments in resonant micro/nanoelectromechanical systems (MEMS/NEMS) and with the promise of monolithic integration on chip [10] , [11] , [12] . Intertwined with miniaturizing sizes, shape engineering and materials innovations in the underlying device structures further add great versatility to these advances. Resonant MEMS/NEMS have already taken a variety of shapes including singly- and doubly-clamped beams [13] , [14] , free–free beams [15] , [16] , nanowires and nanotubes [17] , [18] , stretched nanostrings [19] , square membranes [20] , [21] and circular disks [22] , [23] . These make a fascinating toolbox for exploring various resonance modes and degrees of freedom to enable new functions. Beyond the widely studied fundamental mode, higher-order modes have been pursued in cantilever and beam structures towards multimode sensing of nanoparticles and molecules (for example, simultaneously detecting mass and position of a physisorbed particle on resonator surface) [24] , [25] . Disk resonators are a particularly interesting class among all engineered structures for their ultimate azimuthal symmetry that is also compatible with thin film and planar surface nanomachining processes, much larger capturing areas (for sensing) and much higher stiffness hence operating speed, in comparison with their one-dimensional counterparts (that is, beams and wires) with similar lengths. To date, microdisk resonators have mainly been based on silicon (Si), silica (SiO 2 ) and silicon nitride (SiN) [22] , [23] , [26] , [27] . Silicon carbide (SiC) is a very attractive material for making disk-shaped resonators for its unique characteristics [28] including wide bandgap (~2.3−3.3 eV), transparency from visible to near-infrared, large refractive index (2.64), excellent thermal conductivity (~500 W m − 1 K −1 ), very high elastic modulus ( E Y ~400 GPa) and chemical inertness. Efforts on utilizing some of these properties have already established SiC as a technologically important material for critical applications such as high-temperature electronics [29] and harsh-environment MEMS sensors [30] . The tempting perspective for SiC disk resonators, however, has hitherto been much plagued by difficulties in nanomachining SiC to attain stringent device requirements (for example, a desirable radio-frequency (RF) electrostatic SiC microdisk resonator often requires very high aspect ratio coupling nanogaps and highly doped SiC layers embedded in multilayer processes, which remain very challenging for SiC today). Meantime, although the advantages of disks in area and degrees of freedom (over a beam/wire/string counterpart) promise greater functionalities in multi- and high-mode operations, progresses have been quite limited so far, often due to the lack of highly sensitive readout of high modes: even for beams/cantilevers, mostly only the few lowest modes have been well determined and used [24] , [25] . Fundamental issues such as identification of high modes and mode shapes, mode splitting and coupling and so on demand careful studies before we can rationally exploit them in device applications. In this work we develop a unique SiC microdisk resonator platform that enables highly sensitive optical readout of multimode resonances, up to the ninth mode, with all the modes in the HF band, and with detection down to the fundamental limit of device intrinsic thermal fluctuations, that is, the Brownian motions, in all these modes. Further, we develop microspectroscopy and scanning spectromicroscopy measurement techniques on this SiC microdisk platform and combine them to demonstrate spatial mapping and visualization of these multimode resonances. The multimode mapping then enables deterministic mode recognition and uncovers structural asymmetric effects, while revealing rich multimode resonant characteristics. 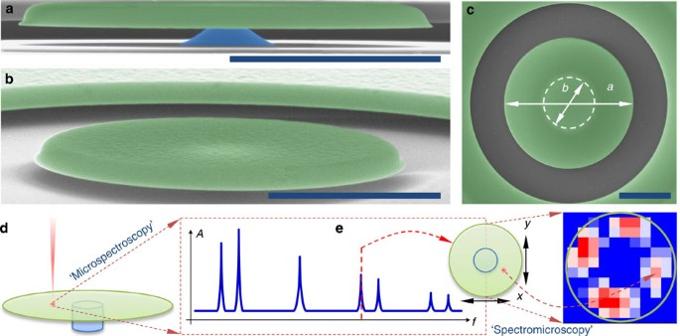Figure 1: SiC microdisk resonators—device structure, fabrication and measurement techniques. (a–c) Side view, aerial view and top view scanning electron micoscope images (colour enhanced) of the 500-nm-thick SiC microdisks supported by underneath 500-nm-thick SiO2pedestal. Scale bars, 5 μm. (d) Illustration of the ‘microspectroscopy’ measurement enabled by the SiC-microdisk optical interferometry, in which wide-range frequency response is obtained while the ~1 μm laser spot is focused on a fixed location. (e) Illustration of the scanning ‘spectromicroscopy’ study where extensive measurements are performed focusing on a specific resonance mode, while the laser spot is scanning over the entire device surface. SiC microdisk fabrication and ultrasensitive motion detection Figure 1a–c demonstrate the SiC microdisks we have developed by nanomachining a 500-nm-thick SiC layer on a 500-nm-thick SiO 2 thermally grown on Si substrate, using a ‘resistless’ process without complicated lithographical steps (see Methods). The SiC-on-SiO 2 technology creates novel centre-anchored circular SiC microdisks featuring a uniform gap defined by the SiO 2 thickness, which is ideal for precision optical interrogation. We have developed an ultrasensitive scanning laser interferometry scheme featuring an ~1 μm spot size on device, capable of directly measuring undriven thermal motions of various devices at room temperature, with fm Hz −1/2 -level displacement sensitivities (see Methods) [31] . In brief, thermodynamic fluctuations agitate a mechanical structure (as dictated by fluctuation-dissipation theorem and equipartition theorem) [32] such that each of the structure’s eigenmodes emerges as a thermomechanical resonance in the frequency-domain noise spectrum, with a displacement noise spectral density of Figure 1: SiC microdisk resonators—device structure, fabrication and measurement techniques. ( a – c ) Side view, aerial view and top view scanning electron micoscope images (colour enhanced) of the 500-nm-thick SiC microdisks supported by underneath 500-nm-thick SiO 2 pedestal. Scale bars, 5 μm. ( d ) Illustration of the ‘microspectroscopy’ measurement enabled by the SiC-microdisk optical interferometry, in which wide-range frequency response is obtained while the ~1 μm laser spot is focused on a fixed location. ( e ) Illustration of the scanning ‘spectromicroscopy’ study where extensive measurements are performed focusing on a specific resonance mode, while the laser spot is scanning over the entire device surface. Full size image where k B , T , ω m , Q , and M eff are the Boltzmann’s constant, temperature, resonance angular frequency of the m th mode, quality factor and modal mass of the eigenmode, respectively. The laser interferometry and optoelectronic readout transduce the displacement-domain noise spectrum into the voltage domain via , where is the interferometric responsivity (displacement to light intensity) and is the optoelectronic responsivity (light intensity to voltage) of the photodetector (PD). The SiC-on-SiO 2 microdisks and their special features, including the uniform 500 nm gap and near-zero absorption at 633 nm in SiC, make it possible to attain exceptionally high transduction responsivities (~20 nV fm −1 ) and displacement sensitivities (~7 fm Hz −1/2 ), which are key to mapping the multimode responses (see Methods and Supplementary Discussion ). We perform two types of measurements ( Fig. 1d,e ): (i) first we measure the wide-range frequency response of all modes while the ~1 μm laser spot is focused on a given location on the device—this is the so-called microspectroscopy measurement ( Fig. 1d ). (ii) For an individual resonance mode of interest, we focus on this resonance and scan the laser spot over the entire device to map out the signal amplitude variations ( Fig. 1e ). We call this scanning spectromicroscopy measurement. In practical scanning, we fix the laser beam path and precisely move the device ( Fig. 1e ) by employing a motorized stage with sub-micron precision, which has the clear advantage of keeping the laser spot undisturbed. 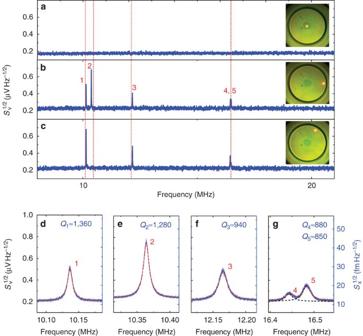Figure 2: Multimode thermomechanical resonances observed in separate microspectroscopic measurements. Wide-range thermomechanical noise spectra measured from a 19.5-μm-diameter SiC microdisk resonator, when the ~1 μm laser spot is focused at the (a) centre of the disk, (b) rim of the disk and (c) another location at the rim, ~60° rotated with respect to the spot inb. Sequence labels for all the observed modes are shown inb. Insets: optical images clearly showing the locations of the laser spot. (d–g) High-spectral-resolution scans of these thermomechanical resonances with extracted quality (Q) factors. Dashed lines are fits to the resonances based on finite-Qharmonic resonator model (equation 1). Multimode mapping and mode recognition Figure 2 demonstrates the microspectroscopy measurements from a representative device (with a disk diameter a =19.5 μm and pedestal diameter b =3.8 μm). We first focus the laser at the centre of the microdisk ( x =0 μm, y =0 μm), right on top of the pedestal ( Fig. 2a ): no resonance is observed as expected. We then move the laser spot to position b ( x =8 μm, y =0 μm) near the rim ( Fig. 2b ), and five resonances become clearly visible, with resonance frequencies in the range of f =10.14 to 16.48 MHz and quality factors Q s≈850−1,360 ( Fig. 2d–g ). At position c ( x =5 μm, y =7 μm), four resonances can be detected ( Fig. 2c ). This clearly demonstrates a probe-position dependence in measuring these multimode resonances. In these measurements, an excellent displacement sensitivity is achieved in the ~5−20 MHz range (see Methods). The sensitivity is set by both the SiC-microdisk interferometry and the optoelectronic transduction downstream; this combination is key to reading out the device's intrinsic thermal motions. Figure 2: Multimode thermomechanical resonances observed in separate microspectroscopic measurements. Wide-range thermomechanical noise spectra measured from a 19.5-μm-diameter SiC microdisk resonator, when the ~1 μm laser spot is focused at the ( a ) centre of the disk, ( b ) rim of the disk and ( c ) another location at the rim, ~60° rotated with respect to the spot in b . Sequence labels for all the observed modes are shown in b . Insets: optical images clearly showing the locations of the laser spot. ( d – g ) High-spectral-resolution scans of these thermomechanical resonances with extracted quality ( Q ) factors. Dashed lines are fits to the resonances based on finite- Q harmonic resonator model (equation 1). Full size image To fully understand and quantitatively demonstrate the position-dependent nature of the multimode resonance spectra, we now focus on measuring the peak amplitude of each of the five resonance modes, while scanning the laser spot throughout the device area (that is, the so-called scanning spectromicroscopy) [33] , [34] . The left panels in Fig. 3a–e present the mode-shape maps measured from all the five resonance modes in Fig. 2 , vividly revealing the shapes and topologies of the undriven Brownian motions of the microdisk. In comparison, the right panels in Fig. 3a–e show the expected resonance mode shapes from finite element modelling (FEM, in COMSOL). We also plot the FEM-computed f -values as dashed vertical lines in Fig. 2a–c . For all the five modes and for both f -values and mode shapes, very good agreement is attained between measured data and simulations. The mode-shape maps also clearly explain the probe-position dependence (observed in Fig. 2a–c ), which originates from the fact that different modes have different nodal diameters/circles where the corresponding resonance amplitudes are vanishing and undetectable. For example, combining Fig. 2c and Fig. 3b , one confirms that position c (inset of Fig. 2c ) is on the nodal diameter of mode 2, thus the absence of this mode in the spectrum of Fig. 2c . 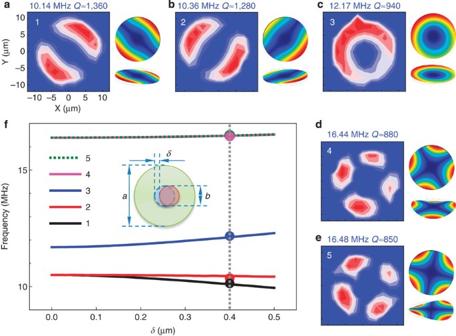Figure 3: Spatial mapping of multimode thermomechanical (Brownian) vibrations of a 500-nm-thick SiC microdisk resonator (a=19.5 μm,b=3.8 μm). The spatial maps are generated by plotting the normalized thermomechanical motion amplitudes obtained from the scanning spectromicroscopy measurements, as functions of the laser spot positions (x,y) (μm). (a–e) Mapping data (on the left of each panel) and FEM computed mode shapes (on the right, both top and aerial views) for resonance modes 1–5 shown inFig. 2, respectively. Red (blue) colour indicates larger (smaller) motion amplitude. (f) Resonance frequencies (f-values) for all these five modes versus the amount of pedestal off-centring (δ). Inset: Definition of device dimensions including the possible off-centringδ(exacerbated, to be visible). Curves: FEM calculation results. Symbols: Measuredf-values of this device. Vertical dashed line indicates the determined pedestal off-centring amount,δ≈0.4 μm. Figure 3: Spatial mapping of multimode thermomechanical (Brownian) vibrations of a 500-nm-thick SiC microdisk resonator ( a =19.5 μm, b =3.8 μm). The spatial maps are generated by plotting the normalized thermomechanical motion amplitudes obtained from the scanning spectromicroscopy measurements, as functions of the laser spot positions ( x , y ) (μm). ( a – e ) Mapping data (on the left of each panel) and FEM computed mode shapes (on the right, both top and aerial views) for resonance modes 1–5 shown in Fig. 2 , respectively. Red (blue) colour indicates larger (smaller) motion amplitude. ( f ) Resonance frequencies ( f -values) for all these five modes versus the amount of pedestal off-centring ( δ ). Inset: Definition of device dimensions including the possible off-centring δ (exacerbated, to be visible). Curves: FEM calculation results. Symbols: Measured f -values of this device. Vertical dashed line indicates the determined pedestal off-centring amount, δ ≈0.4 μm. Full size image The high spectral and spatial resolutions of the scanning spectromicroscopy techniques immediately enable us to unambiguously identify mode sequence and precisely distinguish the split degenerate modes. For a slender-pedestal device as shown in Figs 2 and 3 , in contrast to disk resonators with wider pedestals, the fundamental ‘umbrella’ mode (third peak in Fig. 2b ) is no longer the lowest mode, but instead the ‘wing-wave’ modes (first two peaks in Fig. 2b ) occur at lower frequencies. This ‘mode-crossing’ mechanism is an interesting feature that may be intentionally exploited by tuning device geometry. Shown in Figs 2 and 3 , the measurements reveal that the two theoretically degenerate ‘wing-wave’ modes split in their resonance frequencies ( f 1 =10.14 MHz, Q 1 ≈1,360 and f 2 =10.36 MHz, Q 2 ≈1,280, with Δ f =0.23 MHz, 2.3% of the nominal), as well as the two degenerate ‘quadrantal’ modes ( f 4 =16.44 MHz, Q 4 ≈880 and f 5 =16.48 MHz, Q 5 ≈850), with Δ f =0.04 MHz, 0.24% difference. The spontaneous splitting of degenerate modes, presumably due to subtle asymmetries practically exist in the material and structures (in comparison with ideal, theoretical degeneracy), creates more mode pairs that may have interesting device implications. Identifying structural asymmetry and defects The spatial mapping of the multimode resonances also demonstrates itself as a precise probe for quantitatively revealing asymmetry and structural defects. The measured mode shapes show that due to a slight deviation δ of the pedestal from the exact geometric centre (see Fig. 3f inset), the ‘umbrella’ mode ( Fig. 3c ) no longer has the expected symmetry, but instead exhibits larger amplitude on the opposing side from the pedestal. For the split ‘quadrantal’ modes 4 and 5, the asymmetry due to pedestal off-centring is also evidently visualized in their mapped mode shapes (shown in Fig. 3 ). The measurements also confirm that the ‘wing-wave’ mode with nodal diameter going through the off-centred pedestal, mode 1 ( Fig. 3a ), has lower frequency, as expected from simulations. Exploiting this capability of resolving both f -values and mode shapes for all these modes, we are able to quantitatively determine the extent of asymmetry. Figure 3f shows the FEM calculated f -values of the first five modes for a SiC disk ( a =19.5 μm, b =3.8 μm) with its pedestal deviating from the centre in a range of δ =0−0.5 μm, in comparison with measured data. We find excellent match in both f -values and mode shapes for the five modes all together, with a pedestal off-centring deviation δ =0.4 μm. Asymmetries and structural defects at such sub-micron levels are difficult to observe and quantify using imaging techniques (optical or electron microscopes), but can be precisely determined by the multimode mapping. Visualizing Brownian motions up to the ninth mode We further demonstrate even higher-order multimode mapping for a SiC microdisk with a =29.5 μm and b =7.3 μm ( Fig. 4 ). From wide-range microspectroscopy measurement, nine thermomechanical resonances (labelled 1 to 9) are observed in the HF band. Despite the fact that the higher modes have much smaller thermomechanical motion amplitudes (scale approximately as f −3/2 assuming similar Q s) and therefore are increasingly challenging to detect, our ultrasensitive measurement techniques are capable of directly detecting and profiling the Brownian motions for all the nine flexural modes, with an exceptionally good displacement sensitivity ≈7−9 fm Hz −1/2 in the spectral range of ~5−30 MHz (see plots in Fig. 4a , right axes). 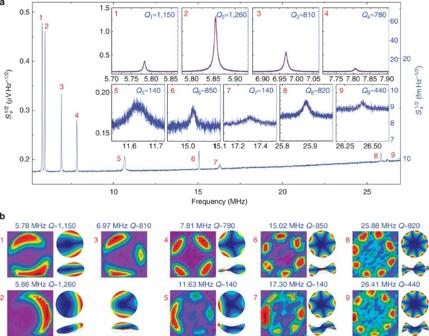Figure 4: Spatial mapping of multimode Brownian motions up to the ninth mode for a SiC microdisk resonator (a=29.5 μm,b=7.3 μm). (a) Wide-range frequency spectrum with nine observed thermomechanical resonance modes. Insets: The nine individual resonances with detailed characteristics, including Brownian motion strength and noise floor in the displacement domain. (b) High-resolution spatial mapping of all the nine modes. Shown for each mode are the experimentally mapped mode shape (on the left of each panel), frequency and quality factor (top), and FEM simulated mode shapes (right, both top and aerial views). Red (blue) colour indicates larger (smaller) motion amplitude in the normalized mode shape maps. Figure 4: Spatial mapping of multimode Brownian motions up to the ninth mode for a SiC microdisk resonator ( a =29.5 μm, b =7.3 μm). ( a ) Wide-range frequency spectrum with nine observed thermomechanical resonance modes. Insets: The nine individual resonances with detailed characteristics, including Brownian motion strength and noise floor in the displacement domain. ( b ) High-resolution spatial mapping of all the nine modes. Shown for each mode are the experimentally mapped mode shape (on the left of each panel), frequency and quality factor (top), and FEM simulated mode shapes (right, both top and aerial views). Red (blue) colour indicates larger (smaller) motion amplitude in the normalized mode shape maps. Full size image Figure 4b shows experimentally mapped mode shapes vis-à-vis FEM simulations for all the nine modes, where we have found (from extensive parametric simulations) that an off-centring of δ =2 μm yields this set of simulated mode shapes that best match the set of mapping results. These highly spatially resolved high-order mode-shape maps again prove powerful and effective in determining mode sequence and revealing effects from device asymmetry. Meantime, we note that the frequency discrepancies of split degenerate modes in Fig. 4 are less uniform than those in Fig. 3 (specifically, 1.4% between 1 and 2, 49% between 4 and 5, 15% for 6 and 7, and 2.0% for 8 and 9), and are difficult to reproduce with the simple model demonstrated in Fig. 3f . This implies second-order effects (such as subtle deviations from circular shape of the pedestal, or disk thickness inhomogeneity) may be superposed to the effects due to simply off-centring the nominally circular pedestal. Multimode resonance frequency scaling We now explore tuning and scaling the frequencies of the multimode resonances via dimension engineering. For centre-clamped disks, the governing equation for the transverse flexural vibrations is [35] , [36] , [37] , [38] where u ( r , θ , t ) is the time-dependent displacement at ( r , θ ), and ρ , E Y , h and ν are the density, Young’s modulus, disk thickness and Poisson’s ratio, respectively. Assuming that the solution takes the form u = U ( r ) sin ( sθ ) sin ( ωt ), with U ( r ) being the radial amplitude profile, s the number of nodal diameters and ω the angular frequency, one then obtains Here is a mode-dependent parameter that can only be determined numerically, and solving λ requires iterative calculation for each given b / a . For example, in the simplest ( s =0, n =0) case ( s , n being index numbers of nodal diameters and nodal circles), by applying the boundary conditions, we can calculate λ 0,0 by solving the determinant equation where J n , Y n ,/ I n , K n are the n th order Bessel functions/modified Bessel functions and η = b / a . For higher modes, it requires solving increasingly complicated equations. Once the solution for λ is found, one can then determine the resonance frequencies using . In practice, even for a single given mode ( s , n ), solving λ s,n for one b / a value requires extensive calculations (with the groups of Bessel functions), and no analytical expression is available for explicitly determining the multimode f -values. Conventionally, results of only very few b / a values on very few modes have been calculated and tabulated in literature [35] , [36] , [37] , [38] . Here, to examine a wide range of device parameters for the multimode resonances, we perform extensive FEM simulations with finely varying dimensions to determine their f -values and mode shapes ( Fig. 5 ), and compare the computation results with experimental data. 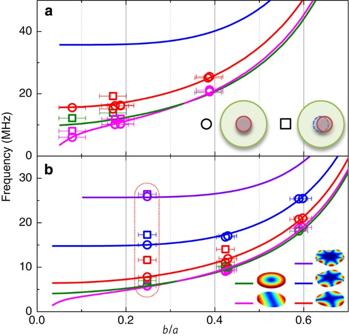Figure 5: Multimode resonance frequency tuning capability by varying pedestal size and disk diameter. Resonance frequencies are plotted as functions ofb/a(the ratio between the pedestal and disk diameters). Data and analysis of multimode resonances scaling versusb/afor (a) six devices witha=19.5 μm andb=1.5, 3.3, 3.4, 3.7, 7.5 and 7.6 μm; and (b) five devices witha=29.5 μm andb=7.3, 12.5, 12.7, 17.4 and 17.6 μm. Curves: FEM computation results of multimode resonance scaling. Symbols: Experimental data. Different colours represent different mode shapes (see bottom legends). Data symbols and computed curves belonging to the same mode are assigned with the same colour. Examples of measured mode shapes demonstrated inFig. 4correspond to the data points inside the dotted line box here. Square symbols indicate resonance modes that appear to be affected by the device asymmetry (see top legends). The error bars for theb/avalues represent the errors in estimating the device sizes, and are 0.03 for the 20-μm disks and 0.02 for the 30-μm devices. Figure 5: Multimode resonance frequency tuning capability by varying pedestal size and disk diameter. Resonance frequencies are plotted as functions of b / a (the ratio between the pedestal and disk diameters). Data and analysis of multimode resonances scaling versus b / a for ( a ) six devices with a =19.5 μm and b =1.5, 3.3, 3.4, 3.7, 7.5 and 7.6 μm; and ( b ) five devices with a =29.5 μm and b =7.3, 12.5, 12.7, 17.4 and 17.6 μm. Curves: FEM computation results of multimode resonance scaling. Symbols: Experimental data. Different colours represent different mode shapes (see bottom legends). Data symbols and computed curves belonging to the same mode are assigned with the same colour. Examples of measured mode shapes demonstrated in Fig. 4 correspond to the data points inside the dotted line box here. Square symbols indicate resonance modes that appear to be affected by the device asymmetry (see top legends). The error bars for the b / a values represent the errors in estimating the device sizes, and are 0.03 for the 20-μm disks and 0.02 for the 30-μm devices. Full size image Figure 5 illustrates the computed curves of f -values scaling with b / a , decorated with experimental data and legends of the corresponding mode shapes from the simulations. Excellent agreement is achieved between the measured and computed f -values. The computed curves show that especially in the vicinity of ‘mode crossing’ (between the first two mode shapes), it might be difficult to determine the mode identification of the individual observed resonances from the f -values alone. Facilitated by the mapped mode shapes, we are able to unambiguously assign each mode in the measured spectrum to a particular mode shape (that is, symbols and curves of the same colour in Fig. 5 have been determined to be from the same mode). These results suggest a dimension-regulated frequency control capability yet to be explored: through careful engineering of the device dimensions, one can not only vary the f -values (the ‘pitches’) but also finely tune the sequence and f -ratios between the different modes (the ‘tones’). Multimode quality ( Q ) factors Furthermore, we investigate the multimode quality ( Q ) factors in addition to tuning and scaling the multimode resonance frequencies. 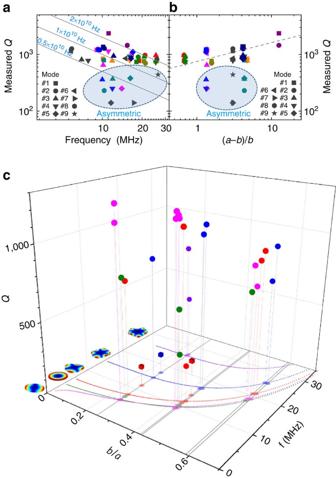Figure 6: Measured quality (Q) factors of multimode SiC microdisk resonators. The measuredQs are plotted against (a)f-values and (b) (a−b)/b, with modes coded in symbol shapes and different devices coded in colours. The shaded regions are the resonance modes that appear to experience more asymmetric effects (for example, exhibiting more asymmetric mode shapes, seeFig. 4). Dashed lines inashow contours of the figure of meritf×Qand the dashed line inbisQ~[(a−b)/b]1/3. (c) MeasuredQs with varying pedestal size (thusb/a) and frequency for five devices all with same diametera=29.5 μm. The projection of this thee-dimensional plot in thef−b/aplane reproducesFig. 5b, with identical colour coding (for all the mode shapes). Cubes (corresponding to squares inFig. 5b) represent the resonant modes experiencing more asymmetric effects. Figure 6a shows the measured Q versus f -values for all the devices measured, with most modes exhibiting the figure-of-merit f × Q >10 10 Hz and the best ones approaching f × Q ≈3 × 10 10 Hz. We notice that, interestingly, in the split degeneration pairs, the one mode with more asymmetric mode shapes often has a lower Q than its conjugate has (for example, in Fig. 4 , mode 5 compared to 4, 7 to 6 and 9 to 8). The disparity in their Q s appears to suggest an intriguing possibility that small structural asymmetries or defects may help amplify the dissipation ( Q −1 ) of the less-favoured mode in the pair. Moreover, as demonstrated in Fig. 6b , we have observed interesting correlation between measured Q s and ( a − b )/ b , ratio between the characteristic lengths of the suspended structure and clamping pedestal. This clearly suggests an intuitive evidence of clamping losses among all the multimode SiC resonators with varying dimensions. Except for the apparently lower Q s from asymmetry-compromised modes in the degenerate pairs, all other measured Q s from multimode resonances align quite well with a power law dissipation Q −1 ~[ b /( a−b )] 1/3 . We find this loss dependence is weaker than the known clamping losses in beam/cantilever structures [39] , where Q −1 ~( w / L ) for out-of-plane flexural modes, with w and L being the clamping width and length of the beam/cantilever, respectively. These evidences for clamping losses and the possibly new power law, together with future experiments at different temperatures (for example, from cryogenic to high temperatures that are achievable for SiC devices, to examine the temperature-dependent Q s), may lead to new studies and guidelines for designing and optimizing the Q s. Figure 6: Measured quality ( Q ) factors of multimode SiC microdisk resonators. The measured Q s are plotted against ( a ) f -values and ( b ) ( a − b )/ b , with modes coded in symbol shapes and different devices coded in colours. The shaded regions are the resonance modes that appear to experience more asymmetric effects (for example, exhibiting more asymmetric mode shapes, see Fig. 4 ). Dashed lines in a show contours of the figure of merit f × Q and the dashed line in b is Q ~[( a − b )/ b ] 1/3 . ( c ) Measured Q s with varying pedestal size (thus b / a ) and frequency for five devices all with same diameter a =29.5 μm. The projection of this thee-dimensional plot in the f−b / a plane reproduces Fig. 5b , with identical colour coding (for all the mode shapes). Cubes (corresponding to squares in Fig. 5b ) represent the resonant modes experiencing more asymmetric effects. Full size image To further demonstrate and analyse the multimode effects on Q s, Fig. 6c plots Q versus multiple device parameters for five devices (with a =29.5 μm and b =7.3, 12.5, 12.7, 17.4 and 17.6 μm). The data show that devices with relatively wider pedestal (larger b ) have less spread in measured Q s, suggesting less effect from pedestal off-centring (that is, δ ≪ b ), such as the device with b / a ≈0.59 and 0.60 in Fig. 6c . For devices with relatively large δ or small b , the asymmetry and imbalance are relatively stronger, causing one of the modes in the degenerate pairs to have a relatively lower Q , as shown in Fig. 6c , by the cube symbols (mode 5 and 7 from the device with b / a ≈0.25, and by mode 5 from the device with b / a ≈0.42). In summary, we have demonstrated multimode SiC microdisk resonators by using a new surface nanomachining process with a 500-nm SiC-on-SiO 2 technology that features a uniform gap and an underneath clamping pedestal with tunable diameter. Along with excellent properties of SiC, this has enabled spectral readout and spatial mapping of the shapes of Brownian motions of the microdisks, up to the ninth mode, by employing scanning interferometry with sub-10 fm Hz −1/2 displacement sensitivity. This study provides deterministic information for identifying the mode sequences in multimode disk resonators, along with key characteristics of the multiple modes that are required for multimode signal processing and sensing [40] . The SiC multimode microdisks will help advance recent attempts towards multimodal sensing of individual adsorbing particles and surface adsorbates phase changes and dynamic fluctuations [24] , [25] , [41] , [42] , with dramatically enhanced capturing surfaces and multi-modalities. The unique transparency of SiC and its near-zero absorption of wide range in visible also make the SiC-on-SiO 2 microdisks an ideal platform for multimodal sensing in liquids [43] , [44] . Further, visualizing the shapes of Brownian motions up to high-order modes help create unprecedented freedom for coupling spatial or topological signatures into fundamental noise processes, which could be of fundamental importance for both classical and quantum-limited measurements (for example, of displacements and forces) [45] , [46] . We have also demonstrated that the multimode mapping is highly responsive to, and offers a new multifold probe for precisely identifying, structural defects such as a sub-500-nm anchor offset. This could be extended to resolving other mesoscopic non-idealities and defects embedded in the devices. Particularly in SiC, defect spin qubits have already emerged as a promising approach towards room-temperature quantum information processing [47] , with unique polytype control capabilities [48] . The spatially mapped SiC multimode resonances down to the Brownian motion limit makes it possible for new exciting experiments on exploring dynamics and propagation of randomly or rationally patterned defects arrays, and coupling defect spin qubits with multiple radio-frequency high- Q mechanical modes. All these enticing interactions enabled by the spectrally and spatially mapped multimode SiC microdisk resonators will engender a plethora of new possibilities for efficiently encoding and transducing information, for sensing and high-security encryption, in both classical and quantum domains. SiC thin film growth and device fabrication The 500-nm SiC layer is grown on SiO 2 by a customized high-throughput low-pressure chemical vapour deposition process on 4-inch wafers, using dichlorosilane (SiH 2 Cl 2 ) and acetylene (C 2 H 2 ) dual precursors at a temperature of T ≈900 °C and pressure of p ≈0.5 Torr, by following methods detailed in previous growth studies [49] . The customized SiC process yields low-stress, high-quality crystalline SiC of the cubic polytype (3C-SiC) with excellent optical, mechanical and thermal properties. SiC film with thickness <500 nm has surface roughness of ~8 nm (Ra) and becomes rougher as thickness further increases. We use focused ion beam (FEI Nova Nanolab 200) to pattern and mill through the SiC layer to define the microdisks with various diameters ( Supplementary Fig. 1 ) and then etch the exposed SiO 2 using hydrofluoric acid. We carefully control the etching time to tune the size of the underneath SiO 2 pedestal that supports the SiC microdisk. This process is ‘resistless’, enabling fabrication of SiC microdisks without complicated lithographical steps. More importantly, this SiC-on-SiO 2 technology creates novel centre-clamped circular SiC microdisks featuring a uniform and smooth air/vacuum gap pre-defined by the thermal SiO 2 thickness, which is critically important for mapping the multimode responses (see Supplementary Discussion ). Measurement system The SiC microdisks are not driven by external excitations and thus only undergo Brownian motions that exhibit multimode thermomechanical resonances. The resonances are measured with a custom-built scanning laser interferometry system ( Supplementary Fig. 2 ) with a spatial resolution of 0.3 μm in the scanning mode. All measurements are done at room temperature under moderate vacuum ( p ≈5 mTorr). A He-Ne laser (633 nm) is focused on SiC microdisk using a 50 × microscope objective, with a spot size of ~1 μm on the device surface. Thermomechanical noise spectral density is recorded with a spectrum analyser (Agilent E4440A). Quantifying noise sources in the measurement The measured noise spectral density in the voltage domain, , includes contribution from all available noise sources: device thermomechanical noise , electrical noise from the PD (including dark current noise from the photodiode, Johnson noise and flicker noise from the transimpedance amplifier and other electrical parts and so on), shot noise (due to the discrete nature of photon), excess laser noise (from the electronic parts and gas in the laser tube) and the noise from the spectrum analyser (that is, the ‘baseline’ noise spectral density when nothing is connected to the input of spectrum analyser). To measure device thermomechanical motion, one needs to observe the targeted on top of the background noise of the entire system (sum of all the other terms—note that the sum is made in the noise power domain, that is, ). It is very important to minimize the background to measure the devices’ thermomechanical motion. 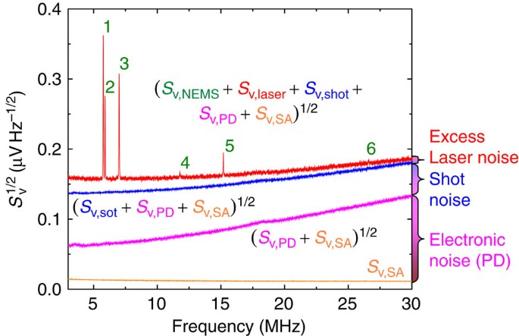Figure 7: Calibration of the noise levels of the measurement system. Orange curve: Spectrum analyser only. Magenta curve: Spectrum analyser+PD (no incident photons). Blue curve: Spectrum analyser+PD (no light)+shot noise (calculation). Red curve: Spectrum analyser+PD+laser (shot noise and electrical noise)+device motion (thermomechanical noise). Labels 1−6 indicate the observed different thermomechanical resonance modes from a typical multimode SiC disk resonator. Figure 7 shows measured noise levels of our system under different configurations. Without any other components connected, the spectrum analyser itself generates a very low noise (orange curve). With the PD (New Focus 1801) connected, and with no incident light (by blocking all incident photons), the noise level (magenta curve) increases noticeably (especially at higher frequencies). This is due to the electrical noise of the PD. When the laser is turned on to measure the thermomechanical motion of device, the noise level further increases with contribution from both shot noise (blue curve) and excess laser noise (red curve). The measured thermomechanical motions exemplify as resonances (labelled with green numbers) on top of the total noise floor. Figure 7: Calibration of the noise levels of the measurement system. Orange curve: Spectrum analyser only. Magenta curve: Spectrum analyser+PD (no incident photons). Blue curve: Spectrum analyser+PD (no light)+shot noise (calculation). Red curve: Spectrum analyser+PD+laser (shot noise and electrical noise)+device motion (thermomechanical noise). Labels 1−6 indicate the observed different thermomechanical resonance modes from a typical multimode SiC disk resonator. Full size image To further understand the contributions from the different noise processes of the laser, here we estimate the shot noise. Its current domain spectral density is where e is electron charge, P in is the incident laser power on the photodiode and is responsivity of the photodiode. In our measurements, P in =290 μW and =0.4 AW −1 (New Focus 1801); thus, we have This is then translated into the voltage domain by the built-in transimpedance amplifier (gain G =40 V mA −1 ): The resulting voltage fluctuations are further divided between the 50 Ω output impedance of the PD and the 50 Ω input impedance of the spectrum analyser. Therefore, its contribution to our measurement is 1.22 × 10 −7 V Hz −1/2 . The blue curve in Fig. 7 shows the calculated contribution from shot noise (on top of the electrical noise from PD and spectrum analyser). From Fig. 7 , it is clear that both electrical noise from the PD ( ) and shot noise ( ) make major contributions to the overall noise floor. The results also show that between these two major noise sources, PD electrical noise (including Johnson and flicker noise) still dominates over the shot noise, especially at higher frequencies. For the measurement system to approach the shot noise limit, one need to further engineer and significantly reduce/minimize the PD noise ( ). In our experiments, the measurement bandwidth is limited by the PDs. To access a larger frequency range, we use two different types of PDs: New Focus 1801 for the range of 25 kHz−125 MHz and New Focus 1601 for 125 MHz−1 GHz. The output from the PDs is recorded with an radiofrequency/microwave spectrum analyser (Agilent E4440A, 3 Hz−26.5 GHz). Interferometric motion transduction The SiC microdisks’ Brownian motions are read out via detecting the motion-modulated interference between the reflections from the SiC disk–vacuum interfaces and the underneath vacuum–Si interface ( Fig. 8a ). The reflectance R of the device (defined as the total reflected light intensity divided by the incidence light intensity) is determined by the interference of the reflected light waves from all the interfaces involved in the device configuration. 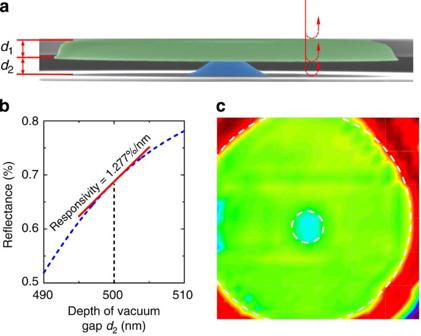Figure 8: SiC microdisk laser interferometric system and calibration of motion transduction/laser heating. (a) Schematic illustrating the multiple reflections of laser beams from all the relevant interfaces. The uniformity of the SiC thickness and vacuum gap ensures a uniform ‘dc’ background or off-resonance baseline throughout the device area, which is key to spatially mapping the multimode motions. (b) Calculated reflectance versus vacuum gap depth. Flexural-mode thermomechanical motion leads to minuscule vertical displacement of SiC microdisk and thus slightly changes the depth of vacuum gap. The slope of the curve at the fabricated gap depth determines the responsivity. (c) Measured reflectance map (in colour scale) of a representative device (its resonance data are shown inFig. 4of the main text), demonstrating uniformity in the measured ‘dc’ and off-resonance background. Dashed circles outline the edges of the disk and the pedestal. Analysis of the multiple reflections inside the device structure gives [50] Figure 8: SiC microdisk laser interferometric system and calibration of motion transduction/laser heating. ( a ) Schematic illustrating the multiple reflections of laser beams from all the relevant interfaces. The uniformity of the SiC thickness and vacuum gap ensures a uniform ‘dc’ background or off-resonance baseline throughout the device area, which is key to spatially mapping the multimode motions. ( b ) Calculated reflectance versus vacuum gap depth. Flexural-mode thermomechanical motion leads to minuscule vertical displacement of SiC microdisk and thus slightly changes the depth of vacuum gap. The slope of the curve at the fabricated gap depth determines the responsivity. ( c ) Measured reflectance map (in colour scale) of a representative device (its resonance data are shown in Fig. 4 of the main text), demonstrating uniformity in the measured ‘dc’ and off-resonance background. Dashed circles outline the edges of the disk and the pedestal. Full size image where r 1 , r 2 and r 3 are the refractive indices at the vacuum–SiC, SiC–vacuum and vacuum–Si interfaces, respectively: Using the absorption coefficient of SiC α =50 cm −1 at 633 nm (ref. 51 ), we obtain the imaginary part of its refractive index κ = αλ /4 π =2.5 × 10 −4 . Combined with its real part [51] , [52] , we have n SiC =2.635–2.5 × 10 −4 i. The refractive index of Si is n Si =3.881–0.019i for 633 nm wavelength. ϕ 1 and ϕ 2 are the corresponding phase shifts: where d 1 is the SiC disk thickness (500 nm), d 2 is the depth of vacuum gap (centred around 500 nm) and λ laser is the laser wavelength (633 nm). Figure 8b presents the calculated reflectance versus vertical displacement for our devices. The slope at d 2 =500 nm gives the ‘displacement to reflectance’ responsivity of the system, . When multiplied by the incident laser intensity, it leads to the ‘displacement to light intensity’ responsivity, , quantifying the variation of interferometric intensity per unit device motion. The reflectance value at d 2 =500 nm determines the ‘dc’ (no device motion) or off-resonance background in the measurement. A uniform d 2 value across the entire device area gives a uniform background (that is, independent of position), which is important for the spatial mapping measurements. Figure 8c plots the off-resonance background (data from measurement of resonance modes 8 and 9 in Fig. 4 ), demonstrating excellent uniformity. Very small lateral distortions visible are due to the minuscule drift and hysteresis in stage position control during the long, intensive scanning measurements. We note that although our device geometry resembles that of an optical cavity, careful measurement and analysis ( Supplement Method ) show that it does not effectively make a high-finesse cavity ( Supplementary Fig. 3 ). Displacement sensitivity calibration We have engineered the system to achieve displacement sensitivities at pm Hz −1/2 to fm Hz −1/2 levels for devices in various materials and structures [31] , by further advancing the interferometry techniques developed during the last decade [53] , [54] , [55] , [56] . To experimentally determine the displacement sensitivity (resolution, or limit of detection for displacement), we first relate the amplitude of the thermomechanical motion to the measured noise level in the spectrum. In the frequency domain, the thermomechanical motion spectral density of any resonance mode m is [32] which at resonance ( ω = ω m ) becomes Here, k B, T , ω m , Q and M eff are the Boltzmann’s constant, temperature, angular resonance frequency, quality factor and the effective mass of this particular mode, respectively. We first calculate the effective mass. For an annular disk clamped at radius r = b /2 and free at r = a /2, the deflection x at a given position ( r , θ ) is [35] where n is number of nodal diameters, b and a are the inner and outer diameters of the disk and A n / B n are parameters depending on n . For example, when n =1, one has and when n =2, Here ν is Poisson’s ratio, and the value of λ is given by where ρ is density and D is flexural rigidity of the disk. Note that for each n , a discrete set of solutions exists for λ (and thus ω m ), corresponding to different s (number of nodal circles, not counting the clamping one at r = b /2) values. Here, we focus on the modes with s =0. Using the normalized deflection , the effective mass coefficient is determined by Using the parameters from the device in Fig. 2 , we obtain , and . For the SiC disk in Fig. 2 with a =19.5 μm, b =3.8 μm, thickness h =500 nm and ρ =3,210 kg m −3 , the effective mass is for n =1. Using this value, we calculate the thermomechanical motion noise spectral density using equation 12 for mode 2 ( n =1) in Fig. 2e of main text ( f =10.36 MHz, Q =1,280), at T =300 K: Assuming the noise processes are uncorrelated, we have . Here is the electronic-domain noise spectral density induced by thermomechanical motion, which is related to the calculated above (equation 19) through the ‘displacement-to-voltage’ responsivity of the SiC-microdisk interferometry system, . The term is the voltage noise floor of the measurement system. Typically, in the 10–60 MHz frequency range (slightly increases with increasing frequency), which sets the off-resonance background ( when ω ≠ ω m ). The displacement sensitivity of the measurement system is defined as and can be estimated using Using the fact that is roughly constant in the frequency range in Fig. 2e , we use the same for both on resonance ( ω = ω m ) and off-resonance ( ω ≠ ω m ). From Fig. 2e , we determine and . Using these numbers with equation 20, we obtain the displacement-domain sensitivity for our experimental setup with this device. For the device with a =29.5 μm, b =7.3 μm and h =500 nm, whose data are presented in Fig. 4 in the main text, for its resonance mode 2 ( f =5.86 MHz, Q =1260), we obtain and the on-resonance thermomechanical motion noise spectral density at T =300 K as: From Fig. 4 , we obtain and near resonance mode 2. The displace sensitivity for this device is therefore Such sensitivities enable the scanning spectromicroscopic measurements to map and visualize the Brownian motions up to the ninth mode. Quantifying the minimal optical absorption and heating A distinct feature of SiC-microdisk laser interferometry is its ultralow optical absorption in a wide range for visible light. For the 633-nm red laser irradiation here, the absorption coefficient for SiC is in the range of α SiC ≈0−50 cm −1 (ref. 51 ). This is very low compared with conventional materials (for example, more than 60 times lower than Si, which has α Si ≈3,200 cm −1 at 633 nm). This ultralow absorption directly translates into a clear advantage of having near-zero parasitic laser heating effects. Below we use α SiC ≈50 cm −1 to estimate the upper limit for any possible heating of SiC microdisks in the experiment. First, using equation 8 with 633 nm laser wavelength, we find that 68.74% of incident light power is reflected from the device structure. The amount absorbed by the Si substrate can then be calculated using [50] where t 1 , t 2 and t 3 are, respectively, the transmission coefficients of vacuum–SiC, SiC–vacuum and vacuum–Si interfaces: From equation 24, we estimate 30.87% of light power is dissipated into the Si substrate. Therefore, only 0.39% of the energy is absorbed by the 500-nm-thick SiC disk. During measurement, the incident laser power is ~2.5 mW, resulting in a maximum possible absorbed power of ~10 μW. Using FEM, we calculate the temperature profile of a device ( a =19.5 μm, b =3.8 μm) under 2.5 mW incident laser (633 nm). The result ( Supplementary Fig. 4 ) shows that the maximum possible temperature increase is negligible (<0.2 K throughout the entire device area). We note that this upper limit estimation of SiC absorption of light and the resulting temperature rise is based on the material properties (absorption coefficients) determined for bulk SiC material. The actual results for chemical vapour deposition-grown film might be different due to factors such as changes in defect structures, surface to volume ratio, surface contaminants and so on. We further experimentally verify the device temperature under 633 nm laser irradiation by employing thermomechanical resonance noise thermometry, which uses the device’s intrinsic thermomechanical noise as a thermometer [32] , [54] , [57] , [58] . Specifically, we compare thermomechanical motion amplitude of the device at different laser power levels. According to equipartition theorem and statistical mechanics, the device temperature is related to the thermomechanical motion amplitude by Here, k eff is the effective spring constant of the resonator and k B is Boltzmann’s constant. Experimentally, we measure the voltage domain noise spectrum, which is related to the displacement domain spectrum through the responsivity . Using this relation, equation 26 becomes The responsivity depends linearly on the incident laser power: , where I is the incident laser power and C is a device-dependent factor. We then normalize the measured signal by dividing it by the incident laser power to compare device temperatures across different levels of incident laser power: Note that for each device, C remains the same for all laser power levels. Using this relation, we verify minimal laser heating effect for the device measured in Supplementary Fig. 5 , for which the normalized thermomechanical resonance amplitude remains the same in the range of 0.186–3.159 mW laser power. Safely assuming a device temperature of 300 K at the lowest laser power level of 0.186 mW laser irradiation, the possible temperature variations throughout the entire range of laser power employed are <5 K, which is within the measurement error bar ( Supplementary Fig. 5a ). It clearly demonstrates that laser heating effect is negligible and the device remains at room temperature. List of all devices and thermomechanical resonances Supplementary Table 1 provides a complete list of all the measured devices and their thermomechanical resonances. Driven resonances and very high f × Q Beyond measuring and spatially mapping the undriven thermomechanical resonances, we have also measured driven responses of our SiC microdisk resonators. We drive the devices opto-thermally by using a radiofrequency/microwave-modulated laser (405 nm) and detect their motions by using the same 633-nm laser interferometry readout system. Supplementary Fig. 6 shows an example of measured driven response from a SiC microdisk device ( t =500 nm, a =19.5 μm, b =3.8 μm) with multiple nanomechanical resonances above 200 MHz. These measured resonance modes in the range of 210–250 MHz (shown in Supplementary Fig. 6 ) all have Q> 10,000. For example, the resonance around 214 MHz has a measured Q of 22,000, giving an excellent figure-of-merit of f × Q ≈5 × 10 12 Hz. How to cite this article: Wang, Z. et al . Spatial mapping of multimode Brownian motions in high-frequency silicon carbide microdisk resonators. Nat. Commun. 5:5158 doi: 10.1038/ncomms6158 (2014).